Characterization of salt-adapted secreted lignocellulolytic enzymes from the mangrove fungusPestalotiopsis sp. Fungi are important for biomass degradation processes in mangrove forests. Given the presence of sea water in these ecosystems, mangrove fungi are adapted to high salinity. Here we isolate Pestalotiopsis sp . NCi6, a halotolerant and lignocellulolytic mangrove fungus of the order Xylariales. We study its lignocellulolytic enzymes and analyse the effects of salinity on its secretomes. De novo transcriptome sequencing and assembly indicate that this fungus possesses of over 400 putative lignocellulolytic enzymes, including a large fraction involved in lignin degradation. Proteomic analyses of the secretomes suggest that the presence of salt modifies lignocellulolytic enzyme composition, with an increase in the secretion of xylanases and cellulases and a decrease in the production of oxidases. As a result, cellulose and hemicellulose hydrolysis is enhanced but lignin breakdown is reduced. This study highlights the adaptation to salt of mangrove fungi and their potential for biotechnological applications. Mangroves are ecosystems commonly found on the coast of tropical and subtropical regions and characterized by the colonisation of the intertidal zone by unique plant species [1] , [2] . Fungi are known colonizers of mangrove forests and the species identified to this day form a large and diversified ecological group, mostly composed of members of the Dikarya subkingdom with a strong dominance of ascomycetes fungi [3] and a limited occurrence of basidiomycetes [4] , [5] . Fungi are able to colonize both the immersed and emerged compartments of the mangrove and they have been identified in the sediments, on floating wood and leaves debris and on the roots, trunks and foliage of the trees [6] , [7] , [8] . Mangroves forests are one of the most productive ecosystems and are characterized by intense carbon processing [9] . Mangrove fungi are thought to have a key role in the detritic food webs and nutrients cycling by contributing to the degradation of particular organic matter into dissolved organic matter, including the very abundant lignocellulosic biomass [10] . In the terrestrial ecosystems, degradation of lignocellulose by fungi has been intensively studied over the last decades [11] . It is based on the secretion of a high number and a broad variety of enzymes that have different and complementary catalytic activities [12] including cellulases, hemicellulases and lignin-modifying enzymes [13] . To this day, however, very little is known about the mechanisms employed by mangrove fungi to breakdown the available lignocellulosic biomass and how their enzymes has adapted to the marine conditions, especially to the presence of high concentrations of salt. It has been shown that several marine ascomycetes encountered in mangrove are capable of wood decay and show cellulose and xylan degradation activities [14] . Furthermore, the study of marine basidiomycetes has revealed that these fungi have the capacity to produce various oxidases such as laccases [15] and manganese peroxidases (MnP), which are among the major lignin-degrading enzymes [16] , [17] . Recently, it was demonstrated that the marine white-rot fungus Phlebia sp. , when grown in presence of 3% sea salt, secretes two different MnP distinct from the one produced in the absence of salt, suggesting that marine fungi may possess sets of alternative lignocellulolytic enzymes adapted to salt [18] . The main goal of the present study is to better understand the influence of salt on the lignocellulolytic enzymes of mangrove fungi, to assess whether different sets of enzymes are secreted in saline and non-saline conditions and if so, how salt affects lignocellulose breakdown. To do so, we isolate several mangrove fungi and screen them in order to select a strain that is both lignocellulolytic and capable of growth in non-saline as well as saline conditions. We select a Xylariales fungus, identified as Pestalotiopsis sp ., and study the enzymatic composition of its secretome when grown on mangrove wood chips with or without salt. As no genomic data are available for this fungus, we first sequence and assemble its transcriptome. This step yield putative transcripts that are functionally annotated. The resulting database is used to annotate the results of a mass spectrometry study of the composition of the secretomes. 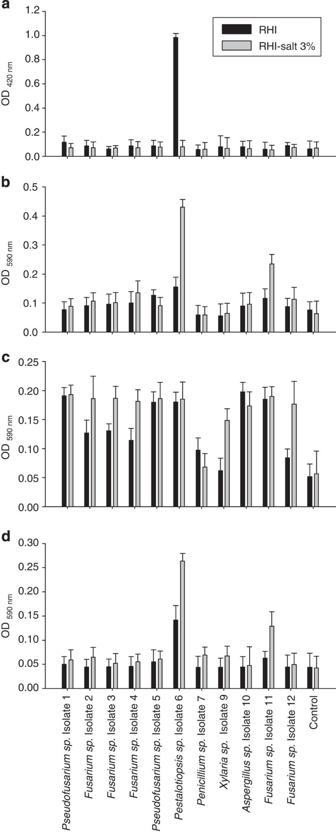Figure 1: Lignocellulolytic activity screening of the isolated mangrove fungi. After 8 days of cultivation in non-saline (RHI) or saline (RHI-sat 3%) conditions, the oxidation of ABTS (a) and the hydrolysis of azo-CM-cellulose (b), azo-carob-galactomannan (c) and azo-xylan (d) in 20 μl of culture supernatant were assessed by spectrophotometry. Each assay was performed twice (two technical replicates) on five biological replicates. Error bars correspond to s.d. Screening of the isolates for lignocellulolytic activities Fourteen fungal strains were isolated to purity from samples collected on various parts of Rhizophora stylosa mangrove trees, exposed cyclically or continually to sea water ( Table 1 ). Of these 14 strains, the isolates 8, 13 and 14 did not exhibit growth when incubated on a solid medium containing R. stylosa wood chips as the main substrate, and thus were removed from the analysis. The 11 remaining strains were screened for their secretion of lignocellulolytic enzymes when grown in a liquid culture medium containing R. stylosa as main substrate (RHI medium: 40 g l −1 R. stylosa wood chips, 1 g l −1 yeast extract, 1 g l −1 malt extract). As these strains were isolated from parts of trees that were exposed to sea water, we conducted the screening in both non-saline and saline (3% w/v sea salt) conditions. The laccase, cellulase, mannanase and xylanase activities in the culture medium were assessed after 8 days ( Fig. 1 ). Laccase activity was only exhibited by the isolate 6 and solely in the absence of salt in the medium. Cellulase activity was detected, albeit at a very low level, for a small number of strains including isolate 4 and 12. Higher levels of cellulase activity were measured for the isolates 6 and 11. For both strains, the activities were, respectively, 2.7 and 2.0 times higher in the presence of salt in the medium. Homogeneous levels of mannanase activity were measured in both medium for all strains, except for isolates 7 and 9, which, respectively, showed overall low activity and low activity in the absence of salt. Finally, the assessment of xylanase activity showed results similar to the cellulase assay, with low values for all strains, except isolates 6 and 11 and with higher activities in the presence of salt (respectively, 1.86 and 2.06 times more). Maximum optical density values for the cellulase, xylanase and mannanase hydrolysis assays were measured by performing an acid hydrolysis (by replacing the biological sample by sulphuric acid at 5% v/v final and heating to 90 °C for an hour). Maximum OD 590 nm was 0.899 (±0.057, s.d. of 5 replicates) for the cellulase assay, 0.275 (±0.041) for the mannanase assay and 0.601 (±0.034) for the xylanase assay. Isolate 6 exhibited the highest activity in all three assays, reaching on average 48, 67 and 44% of the maximum values for the cellulase, mannanase and xylanase assays, respectively. Table 1 List of the fungal strain isolated in this study. Full size table Figure 1: Lignocellulolytic activity screening of the isolated mangrove fungi. After 8 days of cultivation in non-saline (RHI) or saline (RHI-sat 3%) conditions, the oxidation of ABTS ( a ) and the hydrolysis of azo-CM-cellulose ( b ), azo-carob-galactomannan ( c ) and azo-xylan ( d ) in 20 μl of culture supernatant were assessed by spectrophotometry. Each assay was performed twice (two technical replicates) on five biological replicates. Error bars correspond to s.d. Full size image Identification of Pestalotiopsis sp. NCi6 As Isolate 6 exhibited the most diverse set of lignocellulolytic enzymatic activities and showed important variations of these activities depending on the presence of salt, it was selected as a model fungus for this study. Taxonomic identification was performed by studying the conidial characters [19] , [20] ( Supplementary Fig. S1 ) and confirmed that Isolate 6 belongs to the Pestalotiopsis genera. Identification at the species level is uncertain between P. microspora , P. clavispora and P. virgulata . Phylogenetic analysis of the ITS, SSU and beta-tubulin (extracted from the transcriptome, see below) did not resolve this uncertainty (data not shown). Thus, hereafter the isolate 6 is called Pestalotiopsis sp. NCi6 (New Caledonia isolate 6). Effects of salt on the enzymatic activities In order to verify if the variations in enzymatic activities observed for isolate 6 during the screening were the result of a sensibility of the enzymes to salt, the same enzymatic assays as described above were performed but the salinity for the assay was modified. Just before the assays, sea salt was added to the non-saline samples or removed from the saline samples by ultrafiltration ( Fig. 2 ). We observed the same result for every assay: the activities in the non-saline samples was reduced by the addition of salt (laccase: −69±7%; cellulase: −52±4%; mannanase: −61±6%; xylanase: −40±5%) and were reduced in the saline samples by the removal of salt except for laccase (cellulase: −41±4%; mannanase: −55±5%; xylanase: −51±4%). These results indicate that salt has a negative effect on the activity of the enzymes produced in non-saline conditions but has a positive effect on the enzymes produced in saline condition. Thus, it suggests an adaptation of certain enzymes to various levels of salinity and that the variations in activities observed between saline and non-saline conditions are likely to be linked to a modification of the secretome composition. We also monitored the effect of salt on the growth of Pestalotiopsis sp . NCi6 ( Supplementary Fig. S2 ) and observed that the addition of 3% sea salt to the culture medium had no effect. At 6% sea salt, a 2-day-latency phase was observed but growth rate was not significantly affected. This result suggests that Pestalotiopsis sp . NCi6 capacity to metabolize the substrate is not affected by salt. 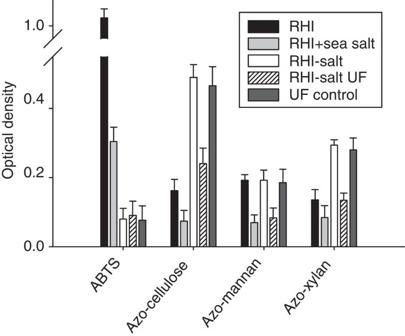Figure 2: Effects of salinity onPestalotiopsis sp. NCi6 enzymatic activities. After 8 days of cultivation in non-saline (RHI) or saline (RHI-Sat 3%) conditions, the oxidation of ABTS and the hydrolysis of azo-CM-cellulose, azo-mannan and azo-xylan by 10 μg of protein were assessed. Sea salt was added to the RHI samples to a final concentration of 3% (RHI+sea salt). Salt concentration was lowered in the RHI-salt 3% samples by ultrafiltration (RHI-salt 3% UF). As a control, the ultrafiltration procedure was performed using a saline buffer (3% sea salt in water) instead of water to check for protein loss induced by the membrane filtration (UF control). Each assay was performed twice (two technical replicates) on five biological replicates. Error bars correspond to s.d. Figure 2: Effects of salinity on Pestalotiopsis sp . NCi6 enzymatic activities. After 8 days of cultivation in non-saline (RHI) or saline (RHI-Sat 3%) conditions, the oxidation of ABTS and the hydrolysis of azo-CM-cellulose, azo-mannan and azo-xylan by 10 μg of protein were assessed. Sea salt was added to the RHI samples to a final concentration of 3% (RHI+sea salt). Salt concentration was lowered in the RHI-salt 3% samples by ultrafiltration (RHI-salt 3% UF). As a control, the ultrafiltration procedure was performed using a saline buffer (3% sea salt in water) instead of water to check for protein loss induced by the membrane filtration (UF control). Each assay was performed twice (two technical replicates) on five biological replicates. Error bars correspond to s.d. Full size image Sequencing and annotation of the transcriptome As no genomic data were available for any members of the Xylariales Order, the possibilities to explore the lignocellulolytic enzymes of Pestalotiopsis sp . NCi6 were limited. Thus, in order to obtain such genomic data, the transcriptome of Pestalotiopsis sp . NCi6 was sequenced and de novo assembled. To capture the largest number of transcripts, a normalized cDNA library was prepared from RNA isolated from pooled samples taken after 2, 4, 6, 8 and 10 days of culture in both non-saline and saline conditions. This library was sequenced using the 454 Titanium platform in a single run from half a picotiter plate. The sequencing run resulted in 676,785 reads, with an average length of 407 nucleotides (N50: 471 nucleotides). After quality check, 602,916 reads (89.1%) were used for assembly using the Roche GS de novo Assembler (Newbler) with default parameters for cDNA. 575,586 reads were assembled in 10,299 isogroups (including 9,559 with a single contig and an average contig content of 1.2). The isogroups are composed of 11,226 isotigs (average length of 1,143 nucleotides, N50 size: 1,379 nucleotides). The assembled isotigs sequences are available in Supplementary Data 1 . De novo functional annotation of the assembled transcriptome was obtained by comparing the isotigs sequences (transcripts) by BlastX against the nr database, resulting in the identification of significant similarities for 8,702 isotigs (77.5%), leaving 2,524 isotigs without any functional information. The BlastX results obtained were used to determine a functional annotation for each sequence using the Blast2GO suite ( Supplementary Methods —annotation of Pestalotiopsis sp . NCi6 transcriptome and Supplementary Figs S3–S6 ). Annotation of the lignocellulolytic enzymes set In order to obtain an expert and accurate annotation of the lignocellulolytic enzymes set present in the transcriptome, the 8,702 isotigs with nr BlastX Hits were compared to the CAZy database ( www.cazy.org ). Overall, 419 isotigs were identified as belonging to one of the CAZy classes ( Fig. 3 , Supplementary Figs S7,S8 and Supplementary Table S1 ). The CAZy annotation identified 238 glycoside hydrolases (GH) distributed in 67 families, including a large number of GH3, GH5, GH61, GH43 with, respectively, 12, 16, 18 and 11 transcripts. The assembled transcriptome also contains 82 glycosyltransferases (GT) distributed in 27 families, 10 polysaccharide lyases (PL) in 3 families, 31 carbohydrate esterases (CE) in 10 families and 22 carbohydrate-binding domains (CBM) in 10 families. Furthermore, 53 potential lignolytic enzymes distributed in 11 families were also identified, including multicopper oxidases, peroxidases, cellobiose dehydrogenases, GMC oxidoreductases and alcohol oxidases. 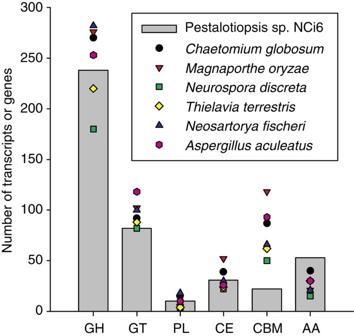Figure 3: Comparison of the CAZomes ofPestalotiopsis sp. NCi6 and of various fungal genomes. The number of putative transcripts annotated in the CAZy classes is reported forPestalotiopsis sp. de novoassembled transcriptome and compared with the number of CAZy genes found in the genomes of various fungi belonging to the Sordariales order (C. globosum,M. oryzae,N. discreta,T. terrestris) and the Eurotiales order (N. fischeri,A. aculeatus). The CAZymes considered here are: the GH, the GT, the PL, the CE, the CBM and the auxiliary activities (AA). Figure 3: Comparison of the CAZomes of Pestalotiopsis sp . NCi6 and of various fungal genomes. The number of putative transcripts annotated in the CAZy classes is reported for Pestalotiopsis sp. de novo assembled transcriptome and compared with the number of CAZy genes found in the genomes of various fungi belonging to the Sordariales order ( C. globosum , M. oryzae , N. discreta , T. terrestris ) and the Eurotiales order ( N. fischeri , A. aculeatus ). The CAZymes considered here are: the GH, the GT, the PL, the CE, the CBM and the auxiliary activities (AA). Full size image Pestalotiopsis sp. NCi6 CAZome (the set of CAZy classified enzymes) was compared with those found in the genomes of the closest fungi publicly available ( Fig. 3 and Supplementary Fig. S8 ). The overall numbers of GH, GT, PL and CE in Pestalotiopsis sp . NCi6, as well as the composition and richness of each family, are comparable to those of several Sordariales and Eurotiales genomes. By contrast, the number of CBM identified in Pestalotiopsis sp. NCi6 transcriptome is noticeably lower than in the other fungi, a decrease that is particularly important for families CBM1, CBM18 and CBM50, corresponding, respectively, to cellulose and chitin-binding proteins. Conversely, Pestalotiopsis sp. NCi6 transcriptome is richer in lignin breakdown enzymes than its counterparts, with an important enrichment of aryl alcohol oxidases. The originality of Pestalotiopsis sp. NCi6 CAZome is apparent in a double-clustering analysis of the number of each CAZy family ( Supplementary Fig. S8 ) where it is segregated from the other species. Analysis of the saline and non-saline secretomes To determine the composition of the secretome produced by Pestalotiopsis sp. NCi6 during its growth on its natural lignocellulosic substrate and how this composition is affected by salt, liquid chromatography-tandem mass spectrometry (LC-MS/MS) proteomic analysis was performed on 8- day-old cultures. Overall, 209 proteins were confidently detected (at least two spectra, Supplementary Methods ) and identified by mass-matching against a database derived from the transcriptome of Pestalotiopsis sp . NCi6 ( Fig. 4 , Supplementary Data 4 ). The GH class accounts for 40% of the secretome with 83 proteins, distributed in 36 families. The most represented families are family GH43 (8 transcripts), family GH61 (7 transcripts), family GH35 (6 transcripts), family GH5 (5 transcripts) and family GH10 (4 transcripts). The second largest group contains 29 proteins corresponding to predicted oxidoreductases with putative lignolytic activities. The secretomes also contain 10 putative CE in six CE families, including four members of family CE12. Finally, the proteomic analysis detected 5 PL, 6 lipases, 9 proteases, 18 unknown proteins and 49 proteins falling in diverse categories such as putative GH not classified by CAZy or various carbohydrate isomerases. 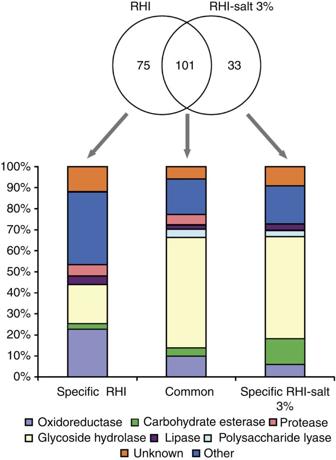Figure 4: Composition of the secretomes ofPestalotiopsis spNCi6 in non-saline and saline conditions. Protein composition of the culture supernatant was assed after 8 days by mass spectrometry. Top: Venn diagram of the number of proteins detected by mass spectrometry and confidently identified in the secretomes ofPestalotiopsis sp. NCi6 when grown in non-saline (RHI) and saline (RHI-salt 3%) conditions. Bottom: putative function of the protein detected specifically in the RHI sample (left), specifically in the RHI-salt 3% sample (left) and common to both samples (middle). Figure 4: Composition of the secretomes of Pestalotiopsis sp NCi6 in non-saline and saline conditions. Protein composition of the culture supernatant was assed after 8 days by mass spectrometry. Top: Venn diagram of the number of proteins detected by mass spectrometry and confidently identified in the secretomes of Pestalotiopsis sp . NCi6 when grown in non-saline (RHI) and saline (RHI-salt 3%) conditions. Bottom: putative function of the protein detected specifically in the RHI sample (left), specifically in the RHI-salt 3% sample (left) and common to both samples (middle). Full size image The secretomes from the two culture conditions differs in size with 176 proteins detected in the RHI samples and 134 in the RHI-salt 3%. One hundred one proteins are common to both secretome, while 75 are specific of the non-saline condition and 33 are specific of the saline condition. These pools of specific proteins differ greatly in terms of composition ( Fig. 4 ). In the saline condition, the proportions of GH (48%) and CE (12%) are several folds higher than in the non-saline condition (respectively, 18% and 2%). Conversely, the proportion of oxidoreductases is strongly reduced in the RHI-salt 3% sample compared with the RHI sample (from 23 to 6%). The composition in GH families is also different between the samples ( Fig. 5 ): the common pool is very diverse (32 families) and mostly comprised of GH5, GH3, GH7, GH43, GH61 and GH10; the pool specific of the RHI sample is composed of 6 families, including enzymes targeting the plant cell wall (GH35 and GH43, both being hemicellulases) and the fungal cell wall (GH72 and GH17); and the pool of GH specific of the RHI-salt 3% is more diverse, with 9 families, and enriched in enzymes targeting cellulose (GH61) and xylan (GH43, GH10, GH30). These specific GH comprise some of the most abundant proteins of the RHI-salt 3% sample, including a GH43 (protein Id: 7189) and GH10 (protein Id: 7566). 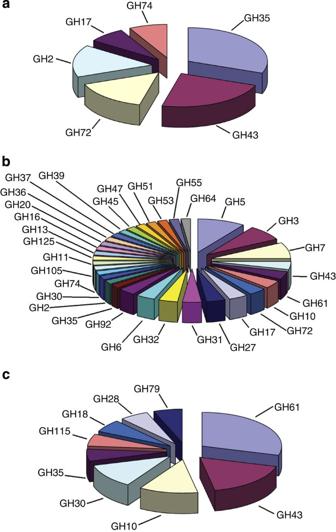Figure 5: Distribution of the GH identified in the secretomes. (a) Fourteen GH identified specifically in the non-saline culture condition. (b) Fifty-three GH identified in both culture conditions. (c) Sixteen GH identified specifically in the saline culture condition. Figure 5: Distribution of the GH identified in the secretomes. ( a ) Fourteen GH identified specifically in the non-saline culture condition. ( b ) Fifty-three GH identified in both culture conditions. ( c ) Sixteen GH identified specifically in the saline culture condition. Full size image The composition in oxidoreductases is also different ( Fig. 6 ): the common pool contains 6 families and is mostly composed of putative FAD-binding oxidoreductases and GMC oxidoreductases; the pool specific of the RHI-salt 3% sample only contains two proteins (including one AA8); and the pool specific of the RHI is the more diverse, with 13 families including GMC oxidoreductases, peroxidases and pyranose oxidases. Several of the most abundant AA detected in the RHI sample are absent from the saline condition, such as an alcohol oxidase (protein Id: 3839), three GMC oxidoreductases (protein Id: 11067, 880 and 938), a glyoxal oxidase (protein Id: 3791) and a peroxidase (protein Id: 2764). 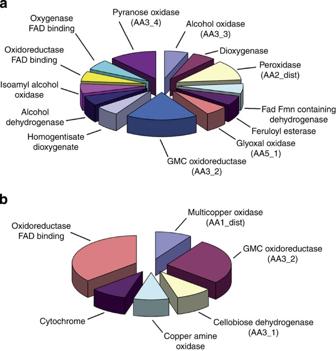Figure 6: Distribution of the oxidoreductases identified in the secretomes. The oxidoreductases category is composed of the proteins identified as AA and of protein annotated as putative oxidoreductase but not referenced in the CAZy AA classification. (a) Seventeen oxidoreductases identified specifically in the non-saline culture condition. (b) Ten oxidoreductases identified in both culture conditions. Only two oxidoreductases have been identified specifically in the saline culture condition: an iron reductase (AA8) and a FAD-binding oxidoreductase. Figure 6: Distribution of the oxidoreductases identified in the secretomes. The oxidoreductases category is composed of the proteins identified as AA and of protein annotated as putative oxidoreductase but not referenced in the CAZy AA classification. ( a ) Seventeen oxidoreductases identified specifically in the non-saline culture condition. ( b ) Ten oxidoreductases identified in both culture conditions. Only two oxidoreductases have been identified specifically in the saline culture condition: an iron reductase (AA8) and a FAD-binding oxidoreductase. Full size image Important rates of lignocellulose mineralization have been demonstrated in mangroves [21] and fungi are thought to be important actors of this process [22] . The lignocellulolytic capabilities of a few mangrove fungi have been highlighted in previous studies [23] and given the influence of sea water on the mangrove ecosystem it is hypothesized that their enzymes may be adapted to tolerate high concentrations of salt. In this study, we screened mangrove fungi for their lignocellulolytic activities when grown on their natural substrate, in the presence or absence of salt. One fungal strain, identified as Pestalotiopsis sp. NCi6, was selected for its wide range of lignocellulolytic activities in both saline and non-saline conditions. Pestalotiopsis sp. NCi6 belongs to the Xylariales Order, a group including a large number of soft-rot and lignolytic fungi [24] . Pestalotiopsis species have mainly been studied for their biotechnological potential as some strains are capable of producing Paclitaxel, a compound used in anticancerous chemotherapies [25] , and various polyketides [26] . Recently, two Pestalotiopsis microspora strains isolated from the Amazonian rainforest showed potential for the biodegradation of polyurethanes plastics [27] . In another study, a strain of Pestalotiopsis isolated from mangrove sediments exhibited laccase activity on a wide range of lignocellulosic substrates [28] . Xylariales in general have gathered a growing interest from the scientific community, as this part of the fungal diversity is still poorly explored and has shown great potential for the discovery of new lignocellulolytic enzymes [23] , [29] , [30] . There is currently no model organism for the study of the Xylariales Order and thus genomic data were unavailable at the beginning of this study. To obtain such large-scale genetic data for the fungus Pestalotiopsis sp. NCi6, we sequenced and de novo assembled its transcriptome rather than its genome. This approach was recently developed to study non-model organism at a fraction of the cost of genome sequencing [31] , [32] . Overall, 11,226 isotigs were assembled in this study. This value is coherent with the number of coding sequences annotated in the genomes of various fungi. For instance, 11,197 gene models were identified in Aspergillus niger ATCC 1015 ( http://genome.jgi.doe.gov/ ) and 11,109 for Magnaporthe grisea [33] . To assess the quality of the assembly, we focused on the results of the CAZy annotation. As the CAZy annotation is based on the recognition of functional domains, backed to a high quality, expertly curated database, it is possible to assess whether an assembled isotig encoding a CAZyme cover the full-length of the functional modules. In our data set, the majority of the isotig were lacking a small fraction at either the N-terminus or the C-terminus. We also noted that a minority (18%) of the CAZy-annotated isotigs are putatively ‘full-length’ as they contain the start codon, preceded by a part of the 5′-UTR, and a complete functional module. As the CAZome richness and composition is partially conserved between species, it is possible to evaluate the completeness of Pestalotiopsis sp. NCi6 CAZome. Here, over 400 putative transcripts have been annotated as CAZymes. This overall value is similar to what has been determined for various species belonging to the Sordariales order (the closest from the Xylariales for which CAZy data are available). For instance, Podospora anserina genome contains 473 CAZymes while 373 CAZymes have been annotated in Neurospora tetrasperma FGSC 2508 genome (Henrissat, unpublished observation). An in depth look at the composition and richness of the different CAZy families suggests that the assembled transcriptome of Pestalotiopsis sp. NCi6 covers a very large portion of the genome. The analysis of the GH set reveals that the distribution at the family level (that is, the number of genes in each GH family) is similar to what is observed in closely related genomes, as the typically enriched families are also enriched in Pestalotiopsis transcriptome. For instance, there are 12 GH3 for an average of 15 in other genomes, 17 GH5 compared with an average of 11 and 13 GH16 for 14 in other fungi. Similar observations can be made for the various GT, PL and CE families. Pestalotiopsis sp. NCi6 showed the ability to grow on a complex lignocellulosic substrate regardless of the presence of high concentrations of salt, but with variations in lignocellulolytic activities. In order to assess the effects of salt on the composition of the secretome, we analysed the protein content of the secretomes by mass spectrometry, and over 200 proteins were confidently detected and identified. As the identification of the proteins is based on mass-matching against the assembled transcriptome, it is possible that a secreted proteins remains undetected because the corresponding transcript is absent from the reference transcriptome, or because the detected protein fragments correspond to a part of the transcript not covered by the isotig. Thus, it is probable that the analysis of the secretome slightly underestimates the enzymatic diversity. Nevertheless, we note that the number of proteins detected is high and similar to other studies. For instance, 242 proteins were identified in the secretome of A. niger when grown on maize bran [34] . In addition to this richness, we also note that the secretome is very diversified. The overall composition of the secretome (that is, the relative abundance of CAZymes, proteases, lipases and so on) is similar to what was observed in that study [34] . The diversity of the proteins found in the non-saline secretome is high and includes a large number of putative enzymes active toward all the parts of the plant cell wall, such as cellulose, hemicellulose, lignin and pectin. The presence of salt in the culture medium resulted in a diminution of the enzymatic diversity, a reduction in lignolytic activity and an increase in hemicellulolytic and cellulolytic activities. The variations in secretome composition appeared to be correlated to the variations in enzymatic activities. For instance, the increase in xylanase and cellulase activities in the saline sample is coupled with the increase in the number of xylanases [35] (GH10, GH30 and GH43) and cellulases [36] (GH61), respectively. Likewise, the complete discontinuation of the ABTS oxidation in presence of salt is clearly coupled to an important decrease of the number and diversity of lignolytic enzymes in the saline secretome. ABTS is usually used as a substrate for laccase activity assay, but can also be easily oxidized by a various oxidative enzymes such as peroxidases [37] , which are also lignolytic enzymes. The reasons explaining the reduction in oxidase abundance are still unclear. For instance, it is possible that the high salinity has an influence on the solubility of lignolysis inductors, thus limiting the expression of the genes encoding lignin degradation enzymes. Recently, laccase, manganese peroxidase and lignin peroxidase activities were reported for several marine fungi when grown under saline conditions [38] . This study suggests that a diverse range of salt-tolerant oxidases exists in the fungal Kingdom, and thus potentially in Pestalotiopsis sp . NCi6. Another noticeable feature of the secretomes is the fact that, for several enzyme families, different proteins are found for the two culture conditions. For instance, multiple GH43 have been identified in Pestalotiopsis sp . NCi6 secretomes, several of which are specific of the saline condition and other of the non-saline condition. As the enzymatic activities are partially lost when the salinity of the assay is modified, we suspect that these proteins correspond to isoenzymes specifically adapted to the salinity. Secretion of isoenzymes as mechanism of adaptation to salt has also been proposed in a previous study [18] , showing that a marine strain of Postia sp . was secreting two MnP in presence of salt to replace the singular MnP produce in absence of salt. Confirming the salt-tolerant or halophilic nature of some of the lignocellulolytic isoenzymes identified in this study of Pestalotiopsis sp. NCi6 would provide further evidences for this model of enzyme replacement. Furthermore, comparing isoenzymes adapted to saline and non-saline conditions would increase our knowledge on the molecular basis of salt-tolerance, leading to the possibility of engineering this characteristic to suit industrial needs. There is currently a growing demand for salt-tolerant lignocellulolytic enzymes to develop various industrial processes, such as biofuels production. The use of ionic liquids to improve lignocellulose solubilisation has been proposed [39] , [40] , [41] , but it requires the discovery of salt-tolerant enzymes [42] , [43] , [44] . Using these enzymes could also allow replacing freshwater by sea water in certain biotechnological applications, thus limiting the consumption of a rare and valuable resource. Currently, only a limited number of salt-tolerant fungal CAZymes have been identified and characterized, but the genome of Pestalotiopsis sp . NCi6 potentially contains several dozens of these enzymes and further, experimental, studies are required to fully explore and exploit this diversity. Sampling, strain isolation and molecular identification Sampling was performed in January 2011 in a small mangrove forest located in the Saint Vincent Bay, Southern Province, New Caledonia (coordinates: −21.934603, 166.078702). The samples were collected from R. stylosa trees on trunks and prop roots bark below maximum sea level. Each sample was enclosed in a plastic bag with 2 ml of distilled water (to maintain humidity) and stored at room temperature in the dark for a week. After incubation, the bags were opened under a laminar air flow cabinet and every visible fungal structure was carefully scrapped with scalpel, inoculated at the centre of a Petri dish containing MY-Agar medium (per litre: 20 g malt extract, 2 g yeast extract, 18 g Bacto Agar) supplemented with chloramphenicol (250 μg ml −1 ) and incubated at 26 °C in the dark. After 3, 5 and 10 days, the plates were observed under a magnifying glass and each fungal strain visible was re-isolated. Isolated strains were maintained on MY-Agar medium at 26 °C in the dark and sub-cultured every 25 days. Preliminary taxonomic identification was performed by sequencing the ITS and SSU rDNA regions (see Supplementary Methods —Molecular identification of the strains). For the strain of interest (Isolate 6, Pestalotiopsis sp. ) identification was confirmed by analysis of morphological traits. Strain cultivation and enzymatic activities screen The fungal strains were screened for growth on a solid medium containing R. stylosa wood as the main nutrients source. To prepare this substrate, two large branches of R. stylosa were collected, had their bark removed, washed with water, dried at 70 °C for 24 h and cut into chips. Chips were grinded using an analytical mill (IKA), the resulting wood fragments were sifted through a metallic mesh (0.8 mm selectivity) and sterilised twice in an autoclave for 1 h at 110 °C. Plates of ‘RHI-Agar’ medium (containing per litre: 18 g Bacto Agar, 1 g malt extract, 1 g yeast extract and 40 g R. stylosa substrate) were inoculated (5 biological replicates) with an agar plug (6 mm diameter) cut from a stock culture and incubated for 30 days. Growth was monitored and only strains able to develop were further considered. Screening for lignocellulolytic activities was performed on liquid cultures in ‘RHI’ medium. Each strain was inoculated in 250 ml baffled Erlenmeyers (five biological replicates) containing 50 ml of medium and incubated at 26 °C in the dark under agitation at 50 r.p.m. (Infors). The inoculum for each Erlenmeyer consisted of two agar plugs (6 mm diameter), cut from the growing edge of a plate stock culture, homogenised in 1 ml of water in Lysing Matrix A tubes with a FastPrep Instrument (MP Biomedicals) at 4 m s −1 for 15 s. Depending on the experiment, the ‘RHI’ medium was supplemented with 3 or 6% (w/v) of sea salt (Sigma-Aldrich). RHI and RHI-salt media are not buffered and pH at inoculation was 5.8 for both. During the growth, pH was slightly increased to an average of 6.3 (±0.2) after 12 days. Enzymatic activities were assessed by collecting a 1-ml sample from each culture every 2 days during 12 days. After centrifugation at 10,000 r.c.f. for 5 min, the supernatant was collected and used in several enzymatic assays (two technical replicates each). Laccase activity was tested by monitoring the oxidation of ABTS (2,2′-azino-bis(3-ethylbenzothiazoline-6-sulphonic acid); Sigma-Aldrich) by adding 20 μl of culture supernatant to 130 μl of 0.1% ABTS in 50 mM citrate-phosphate buffer, pH 5 and measuring the optical density at 420 nm after 30 min of incubation at 26 °C. Endo-1,4-ß- D -glucanase (endo-cellulase), endo-1,4-ß- D -xylanase (endo-xylanase) and endo-1,4-ß- D -mannase (ß-mannanase) activities were assessed by measuring, respectively, the hydrolysis of 1% azo-CM-cellulose, 1% azo-xylan (Birchwood) and 1% azo-carob-galactomannan (Megazyme) in water. Twenty microlitre of culture supernatant were added to 130 μl of azo-substrate solution and incubated 30 min at 26 °C. Three hundred seventy-five microlitre of 95% (v/v) ethanol was then added, and after centrifugation at 5,000 r.c.f. for 10 min, the supernatant was collected and the optical density measured at 590 nm. For the salinity modification experiment, the amount of protein used was standardized at 10 μg for each sample, in a volume of 20 μl. Protein quantification was performed using the Bradford method (Bio-rad Protein Assay) and a BSA standard curve. Salt removal was performed by ultrafiltration using centrifugal concentrating units (Vivaspin 500, Sartorius, PES membranes, 3,000 Da cutoff). The samples were diluted in 1 volume H 2 O and concentrated to initial volume. The process was repeated for five times. To control the impact of the ultrafiltration of enzymatic activities, the same protocol was performed with a saline buffer (MilliQ water containing 3% sea salt) instead of water. Protein loss was assessed by measuring the amount of proteins in the sample before and after the salt removal, using the Bradford method (Bio-rad Protein Assay) and by SDS–PAGE analysis to check for low molecular-weight protein loss and for protein-specific binding to the PES membranes. Growth was monitored every 2 days by measuring the substrate consumption in sacrificed Erlenmeyers. Briefly, the total dry weight of the insoluble part the culture (fungus mycelium and R. stylosa substrate) was measured at the inoculation and after cultivation. Dry weight was determined by filtering the samples with a GF-D filter (Whatman) and by drying the filters at 110 °C until constant weight was reached. RNA extraction, cDNA library construction and sequencing Pestalotiopsis sp . was cultivated in 50 ml of liquid medium ‘RHI’ or ‘RHI-salt 3%’ for 10 days at 26 °C in the dark at 50 r.p.m. For each condition, 15 baffled Erlenmeyers were inoculated with 1 ml of homogenised mycelium (homogenizer: IKA) from a 6-day-old pre-culture grown on liquid malt medium (malt extract 20 g l −1 in water) at 26 °C in the dark. Every second day, three Erlenmeyers for each condition were sacrificed. All the samples were pooled together and centrifuged at 1,000 r.c.f. for 30 s, in order to separate the large wood particles from the lighter mycelium. The supernatant was discarded and the mycelium carefully collected with a spatula. RNA was extracted from the mycelium using the TriZol reagent (Invitrogen) according to the manufacturer’s instructions. After purification, the total RNA qwas quantified using a NanoDrop spectrophotometer (Thermo) and further purified by LiCl precipitation. RNA samples from all the sampling days were pooled and quality was assessed by capillary electrophoresis using a BioAnalyzer (Agilent). The RNA sample was sent to GATC Biotech (Konstanz, Germany) for the subsequent library preparation. Briefly, the mRNA were purified from the total RNA using the Dynabeads mRNA purification kit (Invitrogen) and first strand cDNA were synthesized using random hexamer priming. After ligation of the 454 adapters, the second strand of the cDNA was synthesized and the library was normalized by one cycle of denaturation-reassociation and hydroxyapatite column purification. The purified ss-cDNA were then PCR amplified and the amplicons were size fractionated on gel to select 500–850 bp molecules. The resulting library was sequenced using a GS FLX Titanium and the XLR70 chemistry. Transcriptome assembly and functional annotation After quality check and trimming of the adapter sequences, the sequencing reads were assembled using Roche GS de novo Assembler (Newbler) with the default parameters for cDNA. Functional annotation of the resulting isotigs was performed using the Blast2GO software package ( www.blast2go.com ). BlastX was performed against the NCBI nr database (release of August 2012) with default parameters except for the minimum E -value set at 10 −6 . Blast2GO was also used to map the BlastX results to the Gene Ontology database with default parameters. Annotation of the CAZome (the set of carbohydrate-active enzymes) was performed by translating every isotig presenting a significant BlastX Hit in the frame predicted by the BlastX Best Hit and comparing the amino-acids sequence to the CAZy database (carbohydrate-active enzymes Database; www.cazy.org ). Comparison of the CAZy set of various fungi was performed by double hierarchical clustering using the MEV software ( www.tm4.org/mev/ ). Proteomic analysis of the secretomes Pestalotiopsis sp . was cultivated in 50 ml of liquid medium ‘RHI’ or ‘RHI-salt 3%’ for 10 days at 26 °C in the dark at 50 r.p.m. For each condition, 12 baffled Erlenmeyers were inoculated using the same protocol as the cultures used for the transcriptome preparation. After 8 days of incubation, 6 Erlenmeyers of each condition were sacrificed and pooled. Centrifugation at 10,000 r.c.f. for 15 min was used to separate the mycelium and substrate from the supernatant. The supernatants were incubated 1 h at 4 °C with 5% (w/v) Polyvinylpolypyrrolidone (PVPP) to remove the dissolved tannins produced during fungal growth. PVPP was removed by centrifugation at 10,000 r.c.f. for 5 min. PVPP treatment was repeated twice. Supernatants were then dialysed against 10 volumes of ultra pure water and concentrated using Amicon Poly Ether Sulphone—10 kDa cutoff—and the protein solution was concentrated to a final concentration of 1 μg μl −1 . Protein identification, using LC-MS/MS, was performed at the PAPPSO platform ( http://pappso.inra.fr ), querying trypsic peptides MS/MS data against Pestalotiopsis sp . NCi6 translated transcriptome (all frame, standard genetic code). Proteins identified with at least two unique peptides and a log ( E -value) lower than four were validated. For the detailed LC-MS/MS protocol, see Supplementary Methods —Proteomic analysis of the secretomes. Accession codes: Sequencing reads are available at the EBI Short Reads Archive under the accession number ERP001832. How to cite this article: Arfi, Y. et al . Characterization of salt-adapted secreted lignocellulolytic enzymes from the mangrove fungus Pestalotiopsis sp . Nat. Commun. 4:1810 doi: 10.1038/ncomms2850 (2013).